The HLA-DRβ1 amino acid positions 11–13–26 explain the majority of SLE–MHC associations Genetic association of the major histocompatibility complex (MHC) locus is well established in systemic lupus erythematosus (SLE), but the causal functional variants in this region have not yet been discovered. Here we conduct the first fine-mapping study, which thoroughly investigates the SLE–MHC associations down to the amino acid level of major HLA genes in 5,342 unrelated Korean case–control subjects, taking advantages of HLA imputation with a newly constructed Asian HLA reference panel. The most significant association is mapped to amino acid position 13 of HLA-DRβ1 ( P= 2.48 × 10 −17 ) and its proxy position 11 ( P= 4.15 × 10 −17 ), followed by position 26 in a stepwise conditional analysis ( P= 2.42 × 10 −9 ). Haplotypes defined by amino acid positions 11–13–26 support the reported effects of most classical HLA-DRB1 alleles in Asian and European populations. In conclusion, our study identifies the three amino acid positions at the epitope-binding groove of HLA-DRβ1 that are responsible for most of the association between SLE and MHC. Systemic lupus erythematosus (SLE; MIM 152700) is characterized by chronic and systemic inflammation due to the loss of immune tolerance against nuclear autoantigens. SLE is a polygenic disorder with a genetic heritability of 44−66% (refs 1 , 2 ). To date, ~60 susceptibility loci have been identified in genome-wide and candidate-gene association studies [3] . Among the reported loci, the major histocompatibility complex (MHC) locus showed one of the strongest contributions to SLE risk in multiple populations [3] , [4] . The human leukocyte antigen (HLA) system within the MHC locus on chromosome 6 consists of MHC class I (classical genes: HLA-A , -B and -C ; non-classical genes: HLA-E , -F and -G ), MHC class II (classical genes: HLA-DP , -DQ and -DR ; non-classical HLA genes: HLA-DM and -DO ) and MHC class III (complement and cytokine genes) [5] . Previous association studies have consistently identified the SLE-risk effects of two classical alleles of HLA-DRB1 (*03:01 and *15:01) in both European and Asian ancestries [4] , indicating that the HLA-DR-mediated immune response plays an important role in SLE pathogenesis. Several studies have attempted to dissect the SLE association within the extended MHC locus characterized by a high degree of linkage disequilibrium (LD) and genetic diversity [6] , [7] , [8] , [9] , [10] . Multiple HLA alleles and non-HLA variants in MHC locus have been suggested to have independent SLE-risk effects, as demonstrated by stepwise conditional analysis or HLA allele–allele haplotype analysis to control for the LD effect [6] , [7] , [8] , [9] . However, there were inconsistent observations among the studies in terms of the number and position of independent SLE-risk loci. This inconsistency could possibly result from the complexity of MHC region or low statistical power. Alternatively, another point worth considering is the exclusion of causal functional variants in the previous analyses. Recent studies on HLA associations in other diseases suggested that amino acid positions were the major driver conferring risk for diseases rather than the classical alleles [11] , [12] , [13] . Coding variants in HLA genes are one of the most important factors influencing the activity and specificity of the HLA molecules, but no study has investigated the possible association of amino acids of HLA genes with SLE susceptibility. Because each amino acid residue is typically assigned to multiple classical alleles, an SLE-risk effect at a certain amino acid position would go undetected if only classical alleles and single-nucleotide polymorphisms (SNPs) were assessed. Furthermore, if there is an amino acid position predominantly associated with SLE, the analysis and interpretation of the secondary effect could be misled by conditioning on a false primary effect. Here we perform a fine-mapping analysis on 5,342 unrelated case–control Korean subjects to systematically dissect genetic basis of SLE within the extended MHC region and to assess the contribution of amino acid variants in HLA genes. We identify primary and secondary association signals at amino acid positions 11, 13 and 26 of HLA-DRβ1 at the epitope-binding groove of HLA-DR molecules. These findings will extend the understanding of the HLA association in SLE. Construction of Asian reference panel for HLA imputation We aimed to look at amino acid positions, classical alleles and SNPs simultaneously to define which variation or position is driving SLE. To this end, we applied an imputation method inferring amino acid residues and classical alleles on eight classical HLA genes ( HLA-A , -B , -C , -DPA1 , -DPB1 , -DQA1 , -DQB1 and -DRB1 ) (ref. 5 ) in our Korean study subjects using recently developed SNP2HLA software [14] , [15] . For the accurate imputation for the Korean population, we developed the largest Asian HLA reference panel from two recent HLA reference panels of Korean [16] ( n =413) and Southeast Asian populations [17] , [18] ( n =441). Both the Korean and Southeast Asian HLA reference panels include classical alleles and amino acids of HLA-A , -B , -C , -DPB1 , -DQB1 and -DRB1 and the Southeast HLA reference panel includes additional information of HLA-DPA1 and -DQA1 . Imputation accuracy of the new reference panel was assessed by calculating the concordance rates between genotyped and imputed HLA alleles of 61 HapMap individuals from Chinese from Beijing, China (CHB) and Japanese from Tokyo, Japan (JPT) who carry 64 two-digit and 110 four-digit alleles in six genotyped genes, including HLA-A , -B , -C , -DRB1 , -DQA1 and -DQB1 . 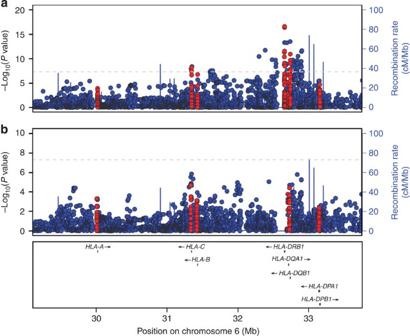Figure 1: Association ofHLA-DRB1with the risk for SLE. The significance levels of all binary-coded markers (blue) and amino acid position (red) in the 5,342 SLE case–control subjects were, respectively, calculated by logistic regression and log-likelihood ratio test and plotted according to their chromosomal position (based on hg 18). (a) The most significant association was observed withinHLA-DRB1in an unconditional analysis adjusting for the top 10 PCs (P=2.48 × 10−17). (b) When the effect of all classical alleles of HLA-DRB1 was additionally adjusted, no signal was found to be associated with SLE susceptibility (P<5.0 × 10−8; gray dashed lines). The new Asian HLA reference panel exhibited average concordance rates of 98.5% at two-digit resolution and 93.2% at four-digit resolution, which were better imputation accuracies than those of the Korean HLA reference panel (95.7%; 91.5%) or Southeast Asian panel (94.1%; 84.7%; Supplementary Table 1 ). At the allele level, the new reference panel showed a high correlation between the imputed and actual dosage (average correlation coefficient r =0.94 for four-digit alleles with frequency ≥0.01; Supplementary Fig. 1 ). We note that we attempted to further merge our new Asian HLA reference panel with a publicly released European HLA reference panel [15] but the overall imputation accuracy became slightly worse when imputing for the East Asian HapMap population using the Asian+European HLA reference panel ( Supplementary Table 1 ). The following association analysis was done with the new Asian HLA reference panel to ensure optimal imputation results. HLA imputation The SNP genotype data of 5,342 unrelated Korean subjects, including 849 SLE cases and 4,493 controls, was obtained from a genome-wide association study (GWAS) data set that had been largely expanded from our previous SLE GWAS [19] ( Supplementary Fig. 2 ). The GWAS data set was filtered using standard quality control criteria based on minor allele frequency, Hardy–Weinberg equilibrium, call rates, heterozygosity rate, population stratification, sex consistency and cryptic relatedness ( Supplementary Fig. 2 ). The study subject was highly homogenous in a principal component (PC) analysis ( Supplementary Fig. 3 ) and a whole-genome association test showed no obvious evidence of systematic bias in our data set ( λ 1,000 =1.04). A total of 86 HLA two-digit alleles, 163 HLA four-digit alleles, 744 HLA amino acid positions and 4,758 MHC SNPs, with frequency (or alternative allele frequency) ≥0.001, were imputed from the genotyped MHC SNPs of the 5,342 study subjects by using the newly developed Asian reference panel. To validate the imputation results, a subset of the study subjects ( n =1,306) was genotyped for four-digit alleles of HLA-DRB1 where the primary association signal could be present. We observed highly reliable concordance rates between the imputed and genotyped alleles (98.6% at two-digit resolution and 95.8% at four-digit resolution) and highly reliable correlation coefficients between imputed and actual dosage (average correlation coefficient r =0.94 for alleles with frequency ≥0.01; Supplementary Fig. 4 ). SLE association at three amino acid positions of HLA-DRβ1 To understand the contribution of variants in the extended MHC locus to SLE susceptibility, we assessed the dosage effect of binary markers (with minor allele frequency ≥1% and imputation quality (Plink INFO value) ≥0.1; encoded as allele 1 and allele 2 or presence and absence) on SLE risk with logistic regression adjusting for the top 10 PCs. In addition, the overall difference of amino acid residues at each amino acid position between case and control groups was examined by a log-likelihood ratio test, comparing the fit between the null model (including the top 10 PCs as predictors) and the full model with amino acid effects. By analysing SLE associations at HLA classical alleles, HLA amino acid positions and SNPs simultaneously in unconditional and conditional analyses, we identified the primary association signal within HLA-DRB1 . When adjusted with all classical alleles of HLA-DRB1 , no additional signal outside HLA-DRB1 passed a genome-wide significance threshold ( P <5 × 10 −8 ) in our subjects ( Fig. 1 ). The most significant association was mapped to the amino acid position 13 of HLA DR chain 1 (HLA-DRβ1), which is located on the epitope-binding groove of HLA-DR ( P= 2.48 × 10 −17 ; Fig. 2a ). This amino acid position better accounted for SLE risk than any other single HLA allele or SNP because the other types of markers were not independently associated with SLE before and after conditioning on the HLA-DRB1 effect. Among two-digit and four-digit classical alleles, the most significant association was observed at two highly correlated alleles ( r 2 =0.94), HLA-DRB1 *15:01 ( P= 5.11 × 10 −14 ) and HLA-DQB1 *06:02 ( P= 3.14 × 10 −14 ), followed by HLA-DQB1*02 ( P= 1.44 × 10 −8 ). Figure 1: Association of HLA-DRB1 with the risk for SLE. The significance levels of all binary-coded markers (blue) and amino acid position (red) in the 5,342 SLE case–control subjects were, respectively, calculated by logistic regression and log-likelihood ratio test and plotted according to their chromosomal position (based on hg 18). ( a ) The most significant association was observed within HLA-DRB1 in an unconditional analysis adjusting for the top 10 PCs ( P= 2.48 × 10 −17 ). ( b ) When the effect of all classical alleles of HLA-DRB1 was additionally adjusted, no signal was found to be associated with SLE susceptibility ( P <5.0 × 10 −8 ; gray dashed lines). 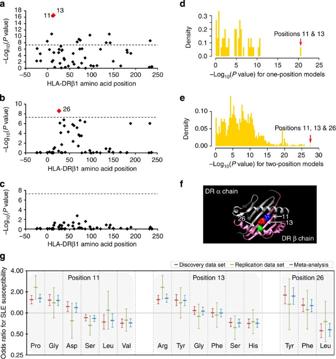Figure 2: Association of HLA-DRβ1 amino acid positions 11, 13 and 26 with risk for SLE. (a) The amino acid position 13 and its correlated position 11 showed the strongest association for risk of SLE in unconditional omnibus tests (n=5,342). (b) The amino acid position 26 was associated after conditioning on the amino acid positions 11 and 13. (c) No amino acid position was associated with the risk of SLE after conditioning on the three positions 11, 13 and 26. (d) APvalue distribution from one-amino acid-position models for SLE risk revealed the best-fit model where the positions 11 and 13 were included. The positions 11 and 13 were considered as a single position due to their tight correlation. (e) Among all possible two-amino acid-position models (n=1,226), the positions 11, 13 and 26 best explained the association betweenHLA-DRB1and SLE. (f) The three amino acid positions 11 (blue), 13 (red) and 26 (green) are on the surface of the epitope-binding groove of HLA-DR (PBD ID: 3pdo). (g) Effect sizes and 95% confidence intervals (error bars) of each residue at the positions 11, 13 and 26 were plotted according to the data sets—discovery data set (n=5,342; red), replication data set (n=496; green), meta-analysis (blue). The effect estimates at the position 26 were calculated in a conditional logistic regression analysis adjusting for the positions 11 and 13. Full size image Figure 2: Association of HLA-DRβ1 amino acid positions 11, 13 and 26 with risk for SLE. ( a ) The amino acid position 13 and its correlated position 11 showed the strongest association for risk of SLE in unconditional omnibus tests ( n =5,342). ( b ) The amino acid position 26 was associated after conditioning on the amino acid positions 11 and 13. ( c ) No amino acid position was associated with the risk of SLE after conditioning on the three positions 11, 13 and 26. ( d ) A P value distribution from one-amino acid-position models for SLE risk revealed the best-fit model where the positions 11 and 13 were included. The positions 11 and 13 were considered as a single position due to their tight correlation. ( e ) Among all possible two-amino acid-position models ( n =1,226), the positions 11, 13 and 26 best explained the association between HLA-DRB1 and SLE. ( f ) The three amino acid positions 11 (blue), 13 (red) and 26 (green) are on the surface of the epitope-binding groove of HLA-DR (PBD ID: 3pdo). ( g ) Effect sizes and 95% confidence intervals (error bars) of each residue at the positions 11, 13 and 26 were plotted according to the data sets—discovery data set ( n =5,342; red), replication data set ( n =496; green), meta-analysis (blue). The effect estimates at the position 26 were calculated in a conditional logistic regression analysis adjusting for the positions 11 and 13. Full size image There are six possible residues (Arg, Tyr, His, Ser, Gly and Phe) at the amino acid position 13. Among them, Arg13 and Tyr13 showed risk effects for SLE (odds ratio (OR)=1.63, 95% confidence interval (CI)=1.45−1.84, P= 1.15 × 10 −15 for Arg13+Tyr13), while His and Ser were protective (OR=0.65, 95% CI=0.58−0.72, P= 4.15 × 10 −14 for His13+Ser13). The other residues Gly13 and Phe13 exhibited no significant effects on SLE risk ( Fig. 2g ). Owing to a tight correlation between positions 11 and 13, a similar level of significance was observed at position 11 ( P= 4.15 × 10 −17 ; Fig. 2a ). Similar to amino acid position 13, increased SLE risk was associated with Pro11 and Gly11 (OR=1.63, 95% CI=1.45−1.84, P= 1.15 × 10 −15 for Pro11+Gly11). It was also noted that these residues perfectly correlated with the SLE-risk residues Arg13 and Tyr13, respectively ( r 2 =1). The SLE-protective residues His13 and Ser13, respectively, showed the best correlations with Val11 ( r 2 =0.90) and Ser 11 ( r 2 =0.41) in the study subjects. Both Val11 and Ser11 were associated with decreased SLE risk (OR=0.69, 95%CI=0.62−0.76, P= 4.81 × 10 −12 for Val11+Ser11). The other residues, Asp11 and Leu11, respectively had modest risk and protective effects ( Fig. 2g ). We note that a conditional analysis adjusting for each of positions 11 and 13 could not statistically distinguish which position is driving SLE ( P value at position 13=2.48 × 10 −5 conditioned on position 11; P value at position 11=4.00 × 10 −5 conditioned on position 13). We then investigated the presence of independent effects that are not accounted by HLA-DRβ1 amino acid positions 11 and 13. In a conditional analysis adjusting for positions 11 and 13, the amino acid position 26 remained significantly associated with SLE susceptibility ( P= 2.42 × 10 −9 ; Fig. 2b ). We surveyed the best-fit model for SLE risk using 1,226 possible combinations of two amino acid positions, assuming the two strongly correlated positions 11 and 13 as a single position. Consistent with the conditional analysis, the amino acid position 26 was found in the best model with the primary-effect positions 11 and 13, although other amino acid positions with weaker significance (for example, position 37 or 74 with omnibus P values ≥1.63 × 10 −7 ) may alternatively explain the risk of SLE due to uncertainty in imputation. The significance level of the two-positions model, including 11, 13 and 26 ( P= 4.59 × 10 −28 ), was highly improved by adding position 26 to the single-position model, which included 11 and 13 ( P= 3.71 × 10 −21 ; Fig. 2d,e ). Importantly, all three positions 11, 13 and 26 are located on the epitope-binding groove of HLA-DR ( Fig. 2f ). A subsequent stepwise conditional analysis showed that there is no additional association signal in coding variants of HLA-DRB1 ( P ≥1.82 × 10 −3 ; Fig. 2c ). We validated SLE association at the HLA-DRβ1 amino acid positions 11 and 13 using independent Korean subjects, including 105 SLE cases and 391 controls. The four-digit alleles of HLA-DRB1 were genotyped and translated to the amino acid residues. Omnibus P values of the amino acid residues at positions 11 and 13 were significant between SLE cases and controls in the replication subjects ( P= 3.27 × 10 −4 for the position 13; P= 5.48 × 10 −4 for the position 11, although the significant levels was slightly weaker than the lowest P value at position −1 ( P= 4.37 × 10 −5 ) probably due to the small size of the replication population. The effect size and direction of each residue at positions 11 and 13 were highly consistent with the original observation in our discovery population ( Fig. 2g ). Position 26 also showed a similar pattern of residue effects when conditioned on the positions 11 and 13. However, the statistical power with the given sample size did not allow us to detect statistical significance at position 26 in the conditional analysis ( Fig. 2g ). By a meta-analysis, we consistently found the primary association at positions 13 and 11 in an unconditional analysis ( P= 9.11 × 10 −22 and P= 3.05 × 10 −20 , respectively) and the secondary association at position 26 in a conditional analysis ( P= 1.40 × 10 −10 ; adjusted with positions 13 and 11). SLE association of HLA-DRβ1 amino acid haplotype We evaluated the associations of amino acid haplotypes defined by the three HLA-DRβ1 amino acid positions 11–13–26. In the Korean subjects, there were 10 haplotypes with frequency ≥0.01 ( Table 1 ). The two well-established SLE-risk HLA-DRB1 alleles *15:01 and *03:01 respectively belonged to two SLE-risk haplotypes, Pro11-Arg13-Phe26 and Ser11-Ser13-Tyr26, among five SLE-risk haplotypes. In addition, our haplotype association results further suggested SLE-risk or SLE-protective roles for classical alleles based on the effect estimates of each amino acid haplotype. The effect directions of most classical alleles, such as *01:01, *04, *07:01, *08, *09:01, *11, *13 and *14, have been consistently observed in previous Asian studies [20] , [21] , [22] . Table 1 Association of the HLA-DR β 1 amino acid haplotype 11–13–26 with susceptibility to SLE. Full size table We further evaluated if the effect sizes of the amino acid haplotypes are concordant with the previously reported effect sizes for classical alleles. The observed effect size of each amino acid haplotype was compared with published results from the largest Asian study [20] investigating the association of classical HLA-DRB1 alleles with SLE susceptibility using 1,697 Japanese case–control subjects. In the Japanese study, seven common haplotypes were present based on the frequency and number of HLA-DRB1 classical alleles. When we calculated crude ORs of each haplotype for SLE risk from the raw count numbers of classical alleles in the Japanese study, a highly correlated trend was observed between the haplotype effect sizes in our study and the Japanese study ( r =0.83; Supplementary Fig. 5 ). In addition, we compared our results with the European haplotype effect sizes derived from the reported association results for classical HLA-DRB1 alleles in the largest European case–control study [9] . The direction of each haplotype effect in the Korean and European populations was the same for most haplotypes and effect size was moderately correlated ( r =0.63; Supplementary Fig. 6 ). Among the 10 observed haplotypes, the haplotype Gly11-Tyr13-Phe26, corresponding to HLA-DRB1 *07:01, was highly distinct between ancestries (OR=1.51, 95% CI=1.26–1.82 in Korean and OR=0.75, 95% CI=0.69–0.82 in European). It might mean that the allele is a functional variant having different effect on SLE in different populations. Alternatively, this ethnic heterogeneity between the Asian and European ancestries for this single haplotype may indicate the presence of additional or unique independent effects in HLA genes and elsewhere within the MHC in the Asian or European populations. We note that the risk effect of HLA-DRB1 *07:01 has been reported in another Asian study using Malay case–control subjects [22] ; however, there was no other study that examined the SLE association of *07:01 in Asian populations due to the low frequency of the *07:01 allele and small sample sizes. When the Gly11-Tyr13-Phe26 haplotype was excluded from the comparison of haplotype effects between the Asian and European data sets, the overall correlation was highly improved ( r =0.82). Distinct residue effects in SLE versus other diseases Since there was notable disease pleiotropy at the HLA-DRβ1 amino acid positions 11 and 13 to other diseases such as rheumatoid arthritis and follicular lymphoma [11] , [12] , [13] , [18] , we further investigated residue effects of these positions on different disease phenotypes. As expected, the residue effects were unique and not correlated between SLE and the two unrelated diseases ( Supplementary Fig. 7 ). Especially, most residues had opposite effects in SLE and rheumatoid arthritis, which was expected based on the previously reported association results of classical HLA-DRB1 alleles in the diseases (discordance P ≤4.78 × 10 −8 ). Our SLE–MHC association study is the first fine-mapping study that thoroughly investigated the associations down to the amino acid level. There are several important points in our case–control association study. First we addressed the effect of coding variants in major HLA genes on SLE risk and identified the predominant association at the amino acid positions 11 and 13 of HLA-DRβ1. Their SLE-risk effects and significance levels were very similar due to a high degree of LD between them. Their functional effects are also expected to be similar because both positions are located on the HLA-DR epitope-binding groove. The exact position with the primary causal effect might be further identified by dissecting the associations using a large subject populations with a relatively weak LD between the two positions or by testing the functional effect of the recombinant HLA-DRβ1 in presenting lupus autoantigens and interacting with CD4+ T cells. In another point of view, it is also possible that the two (or more) amino acid positions cooperatively make a pathogenic structure at the HLA-DRβ1 epitope-binding groove in SLE. In fact, the amino acid properties at positions 11 and 13, such as size, hydrophobicity and polarity, were not correlated with their SLE-risk effects. Thus, the functional role of the amino acid residues at these positions might not only determine their own properties but also cooperatively influence the global structure and context of the HLA DR epitope-binding groove and how HLA-DR binds to autoantigens and T-cell receptors. Second, we found the second independent effect at the amino acid position 26 of HLA-DRβ1 in stepwise conditional analysis. The position 26 significantly improved the SLE-risk model in our data set better than the other positions. However, we do not rule out the possibility that alternative amino acid position could be SLE risk because of the small gap of association P values between positions 26 ( P= 2.42 × 10 −9 ) and other positions ( P ≥1.63 × 10 −7 ). The amino acid haplotype model consisting of positions 11, 13 and 26 for SLE risk explained the association between MHC and SLE risk well, and was consistent to the reported effects of classical alleles for both Asian and Europeans. Our amino acid model was not only parsimonious but also allowed easy cross-population analysis. In 2012, the largest and most recent European SLE fine-mapping analysis on classical alleles and SNPs (but not HLA amino acids) pinpointed HLA-DRB1 *03:01, HLA-DRB1 *08:01 and HLA-DQA1 *01:02 in their best disease model [9] . However, this model was not applicable to Asian populations where the frequency of HLA-DRB1 *03:01 and HLA-DRB1 *08:01 is low or very rare (2.0% and 0.0% in Korean, respectively). In an unconditional analysis of our Korean data set, the observed statistical significance for SLE association was P= 0.02 at HLA-DRB1 *03:01 and P= 0.07 at HLA-DQA1 *01:02 possibly due to low frequencies. In contrast, the amino acid haplotype model was consistent to previously reported effects of classical alleles of HLA-DRB1 in this European population study ( Supplementary Fig. 6 ) as well as other Asian population studies ( Supplementary Fig. 5 ) [9] , [20] , [21] , [22] . In addition, we note that SLE associations at several reported SLE-risk SNPs listed in the NHGRI GWAS Catalog [23] and two independent SLE-risk SNPs in the largest fine-mapping study [9] were much weaker than that at the amino acid positions during the stepwise conditional analysis. Some of these SNPs were not common in the Korean subjects. Third, we constructed the largest Asian reference panel from two previous Asian reference panels [16] , [17] , [18] for fine-mapping MHC association. The new ethnicity-matched HLA reference panel gave us better imputation accuracy than each separate of the panels, although association results were substantially the same regardless of which reference panel we used. Fourth, given our sample size, our study did not have enough statistical power to provide a clear picture of independent effects outside of HLA-DRB1 . We observed some suggestive associations near HLA-B and -C and non-HLA genes ( P ≥1.37 × 10 −6 ) after conditioning on all HLA-DRB1 signals. This observation could be consistent with other fine-mapping studies that showed evidence of multiple independent associations in the MHC region [6] , [7] , [8] , [9] . Therefore, in the future, it is important to expand the same fine-mapping study on HLA alleles, HLA amino acids and SNPs with a larger sample size and multiple ancestral samples. In summary, we demonstrated the new amino acid haplotype model for SLE risk, taking advantage of imputation of functional coding variants in major HLA genes. The haplotype model implicates a critical role for the three amino acid positions on the epitope-binding groove of HLA-DR molecules in conferring risk for SLE. Ethics This study was approved by institutional review boards at Hanyang University and Korea National Institute of Health. All the enroled subjects provided written informed consent for study participation. Study subjects, genotyping and quality control A total of 5,342 unrelated Korean subjects participated in this study, consisting of 849 SLE cases and 4,493 controls recruited from Hanyang University Hospital for Rheumatic Diseases (Seoul, South Korea) and Korea National Institute of Health (Osong, Korea). The SLE patients fulfilled more than four of the 11 criteria for the 1997 American College of Rheumatology [24] for the classification of SLE. Genome-wide SNPs of 4,188 case–control individuals (SLE data set #1) were genotyped using 1M Illumina Omni arrays and SNP data of 1,154 independent case–control individuals (SLE data set #2) was retrieved in our past SLE GWAS [19] ( Supplementary Fig. 2 ). We filtered out individuals with low call rate in each data set (<0.98), sex inconsistency between subject-reported and genetic sex, and cryptic relatedness within and between the data sets (duplicates and cryptic first degree relatives). For each data set, SNPs with poor quality were removed if they show low call rate (< 0.98), Hardy–Weinberg disequilibrium ( P <5 × 10 −7 ), rare minor allele (≤ 2 alleles) or significant difference of missing rates between case and control group ( P <0.05). We obtained the top 10 PCs after merging the two data sets and removed outliers with population stratification (>10 s.d. from 10 PCs; Supplementary Fig. 3 ). The sample size-adjusted inflation factor ( λ 1,000 ) was calculated from the 90% bottom SNPs in the meta-analysis results of logistic regression for each case–control data set. Asian reference panel for HLA imputation To maximize the imputation accuracy, we combined two independent Asian reference panels—Korean panel [16] ( n =413 subjects) and Southeast Asian panel [17] , [18] ( n =441 subjects; Singapore Chinese+Southern Han Chinese+Southeast Asian Malay+Tamil Indian). We obtained the raw genotype data of classical HLA alleles and SNPs, spanning the extended MHC region (25–35 Mbp at chromosome 6, hg 18), which were used to construct each reference panel. All genotype data from the two data sets were merged as a single data set after excluding the SNPs that were not present in both data sets ( n =5,911 SNPs in Korean panel; n =6,989 SNPs in Southeast panel; n =4,766 SNPs in both panels). The amino acid residues of each HLA genes were translated based on the known amino acid sequences of classical alleles of HLA-A , -B , -C , -DPA1 , -DPB1 , -DQA1 , -DQB1 and -DRB1 in the IMGT/HLA database [25] . All information about the SNPs, amino acid residues and two-digit and four-digit HLA alleles were encoded as binary variables and phased by Beagle 3.0.4 imputation program [14] powered by SNP2HLA method [15] with some modifications. Evaluation of Asian reference panel We directly compared the imputed and genotyped results for classical HLA alleles using independent data sets to assess the imputation accuracy of reference panels. We imputed the HLA alleles from the SNP-only data of CHB and JPT. The dense SNP genotypes of the East Asian HapMap subjects were extracted from the HapMap3 r2 database ( http://hapmap.ncbi.nlm.nih.gov/cgi-perl/gbrowse/hapmap3r2_B36/ ). Information about classical alleles of HLA-A , -B , -C , -DQA1 , -DQB1 and -DRB1 in the HapMap subjects was retrieved from two independent studies [10] , [26] . The HapMap subjects with discordant HLA alleles in the two studies were removed from the evaluation. At the gene level, concordance rates between imputed and genotyped classical alleles were calculated for each HLA gene. At the allele level, Pearson’s correlation coefficients between imputed and actual dosage were calculated to evaluate the imputation accuracy. HLA imputation We extracted SNP genotypes within the extended MHC region ( n =4,728 SNPs in SLE data set #1 and n =2,222 SNPs in SLE data set #2) and imputed classical HLA alleles, HLA amino acid residues and untyped SNPs from each data set by using the new Asian reference panel and SNP2HLA [15] ( Supplementary Fig. 1 ). Imputation accuracy was validated by direct comparison between imputed and genotyped results of HLA-DRB1 alleles for 1,306 study subjects consisting of 794 cases and 512 controls. Four-digit classical HLA-DRB1 alleles of the subjects were genotyped by using a WAKFlow HLA typing kit (Hiroshima, Japan). Association analysis We obtained dosage values of imputed markers encoded as (1) allele 1 and allele 2 for biallelic markers (for example, two-allele SNPs, two-residue amino acid positions) or (2) presence and absence of each allele of multi-allelic (≥ 3 alleles) markers (for example, multi-residue amino acid positions, two-digit and four-digit classical HLA alleles). SLE association of the imputed dosage of each marker with minor allele frequency of ≥1% and imputation quality (PLINK INFO) of ≥0.1 was examined by logistic regression including the top ten PC covariates obtained from the merged GWAS data set to adjust for potential population substructure. Applying PCs was considered helpful in our association tests, because the original inflation factor ( λ =1.06; λ 1,000 =1.04) from genome-wide association tests became slightly improved ( λ =1.05; λ 1,000 =1.03). A log-likelihood ratio test, estimating log-likelihood difference due to the effect of m residues at a single amino acid position, was used to evaluate SLE association at an amino acid position. The full logistic model included m−1 residues (excluding the most frequent residue because of colinearity among the m residues) and 10 PCs as predictors for SLE risk. The nested null model only included the PCs. Stepwise conditional analysis was performed to find additional markers with independent SLE-risk effect by adding the identified markers as covariates in logistic regression. We obtained fully phased haplotypes across the extended MHC from the imputed data and extracted the haplotypes defined from HLA-DRβ1 amino acid positions 11, 13 and 26. Haplotype-specific OR of having SLE was calculated for each haplotype versus the other haplotypes by logistic regression adjusting for the top 10 PCs. Replication subjects and genotyping Independent Korean case–control individuals (105 SLE cases and 391 controls) were recruited as replication subjects to validate the association of HLA-DRβ1 amino acid positions 11, 13 and 26 with SLE susceptibility. We genotyped four-digit alleles of HLA-DRB1 in the replication subjects by using a WAKFlow HLA typing kit (Hiroshima, Japan). The amino acid sequence was constructed from the known amino acid sequences of classical HLA-DRB1 alleles. The SLE patients met the 1997 American College of Rheumatology criteria [24] for the classification of SLE. The replication study was approved by the institutional review board of Hanyang University Hospital for Rheumatic Diseases (Seoul, South Korea). Comparison of residue effects between diseases HLA-DRβ1 amino acid positions 11 and 13 have shown the most significant association in SLE and rheumatoid arthritis. We assessed how discordant the effect sizes of each residue are between the SLE and rheumatoid arthritis. There were six different residues at each position. We calculated multivariate betas and s.e. for each residue against a reference residue (Pro11 and Phe13) from our data set and original rheumatoid arthritis data sets [11] , [13] , [18] and tested the discordance of effect sizes between the diseases using the following statistic: where S m and R m are multivariate betas of the m -th residue among the five residues (=6 residues—1 reference residue) at position 11 or 13 in SLE and rheumatoid arthritis, respectively. SV m and RV m are the variances for the betas of the same residues in SLE and rheumatoid arthritis, respectively. Discordance P value was calculated from this statistic that follows χ 2 distributed with five degrees of freedom under the null. How to cite this article: Kim, K. et al . The HLA-DRβ1 amino acid positions 11–13–26 explain the majority of SLE–MHC associations. Nat. Commun. 5:5902 doi: 10.1038/ncomms6902 (2014).